Gradient area-selective deposition for seamless gap-filling in 3D nanostructures through surface chemical reactivity control The integration of bottom-up fabrication techniques and top-down methods can overcome current limits in nanofabrication. For such integration, we propose a gradient area-selective deposition using atomic layer deposition to overcome the inherent limitation of 3D nanofabrication and demonstrate the applicability of the proposed method toward large-scale production of materials. Cp(CH 3 ) 5 Ti(OMe) 3 is used as a molecular surface inhibitor to prevent the growth of TiO 2 film in the next atomic layer deposition process. Cp(CH 3 ) 5 Ti(OMe) 3 adsorption was controlled gradually in a 3D nanoscale hole to achieve gradient TiO 2 growth. This resulted in the formation of perfectly seamless TiO 2 films with a high-aspect-ratio hole structure. The experimental results were consistent with theoretical calculations based on density functional theory, Monte Carlo simulation, and the Johnson-Mehl-Avrami-Kolmogorov model. Since the gradient area-selective deposition TiO 2 film formation is based on the fundamentals of molecular chemical and physical behaviours, this approach can be applied to other material systems in atomic layer deposition. Decades ago, top-down and bottom-up approaches were competitively studied for next-generation nanoscale fabrication. The top-down approach, which is primarily used for the nanofabrication of Si devices using photolithography and etching, has been recently used to fabricate 3D nanostructures, such as nanowires and nanodots, which were previously only obtainable through the bottom-up approach. The top-down approach also facilitates large-scale manufacturing, which has allowed this approach to dominate the current nanofabrication technology. Top-down-approach-based nanofabrication is essential for the construction of modern Si electronics and other devices, such as bio-medical and energy devices. In addition, many challenges that limit top-down-approach-based nanofabrication have been resolved by realising an integrated approach incorporating the bottom-up technology. An example of such an integrated approach is area-selective deposition (ASD) that is based on surface chemical reactivity control. Atomic layer deposition (ALD) enables nanoscale precise thickness control, excellent uniformity and conformality because of the unique surface self-saturated reactions of precursors and counter-reactants [1] , [2] , [3] . Because ALD allows strong surface-dependent growth, a film could be selectively deposited on a specific area to achieve chemical reactivity control. Self-assembled monolayers, organic molecules, polymers and ALD precursors have been introduced to inhibit or promote the surface chemical reactivity of ASD-grown films [4] , [5] , [6] , [7] . An inhibitor selectively adsorbs on a specific surface and inhibits the subsequent ALD growth on the surface only, allowing bottom patterns to transfer to upper patterns through ASD. For example, in our previous study [8] , ASD was conducted using a Si precursor inhibitor that was previously used for the ALD of SiO 2 . The study highlighted that the Si precursor inhibitors selectively adsorbed on a OH-terminated SiO 2 surface but not on a H-terminated Si surface, inhibiting the growth of Pt and Ru ALD. Until now, most ASD-based research has focused on the selective growth between two different surfaces such as SiO 2 /Si, SiO 2 /Cu and SiO 2 /HfO 2 for expanding the application scope of ASD in material fabrication and on the adsorption selectivity of inhibitors [8] , [9] , [10] , [11] , [12] . If the growth selectivity in ASD can be controlled using other factors, such as the geometry of nanopatterns, but not by surface termination, then ASD can be extended to other bottom-up-approach-based applications to overcome the limits impeding nanofabrication. Isotropic growth is the main advantage of ALD; however, such growth induces the negative side effect of seam and void formation in high-aspect-ratio 3D structures such as holes and trenches [13] . As the number of ALD cycles increases, structure openings become closed (pinch-off) at a certain film thickness, forming voids or seams along the centreline as shown in Fig. 1a . The seams and voids are unavoidable critical defects formed during nanofabrication; they degrade device performance, electrical conductivity and thermal or mechanical properties [14] , [15] , [16] . To avoid seam formation, anisotropic growth inside the structure, like V-shaped growth, is required but cannot be achieved from the isotropic growth during ALD (Fig. 1b ) [14] . Fig. 1: Schematic illustrations of ASD processes for seamless gap-filling. a Typical ALD process. b ALD process for V-shaped growth. c The proposed gradient ASD process using an inhibitor. Full size image Seamless deposition of TiO 2 in 3D nanostructures is essential for optical device applications, such as the fabrication of meta-surfaces [17] , [18] , but there is no proper deposition method to realize it [19] , [20] . In this study, we introduce a process of gradient ASD of a TiO 2 film that allows seamless gap-filling; the process is illustrated in Fig. 1c . Through ALD, a TiO 2 film is deposited on high-aspect-ratio (AR) hole patterns; a Ti inhibitor layer is then adsorbed onto this TiO 2 film. The adsorption densities of the inhibitor vary depending on the geometrical positions and induce different blocking properties in the inhibitor. This causes ALD-grown TiO 2 films to grow anisotropically, resulting in gap-filling without seam formation and realising the above-mentioned objective of the proposed gradient ASD concept. To inhibit TiO 2 growth, herein, a Ti inhibitor is introduced, namely, trimethoxy-(pentamethylcyclopentadienyl)-titanium(IV) [TMPMCT], which was originally developed as a Ti precursor for ALD TiO 2 . TMPMCT-inhibited film growth and seamless gap-filling were investigated using various experimental and theoretical methods, including density functional theory (DFT) calculation, Monte Carlo (MC) simulation and the Johnson–Mehl–Avrami–Kolmogorov (JMAK) model. Initial experiments of gradient ASD were demonstrated in a lab-scale ALD system, and its wafer-scale demonstration was performed in a production-scale spatial-divided ALD system. Based on this research, we believe that the proposed approach can be applied for the ALD-assisted fabrication of other material systems. Previous reports suggest that TMPMCT is only oxidised by reactive oxidants, such as ozone and O 2 plasma [21] , [22] , but not by H 2 O [23] , [24] . Thus, if TMPMCT covers a surface before an ALD process using a H 2 O counter-reactant, TMPMCT could inhibit the subsequent ALD growth by assuming no reaction between TMPMCT and the ALD precursor. This study used TMPMCT to inhibit subsequent TiO 2 ALD using a tetrakis(dimethylamido)titanium (TDMAT) precursor and a H 2 O counter-reactant and investigated the adsorption stability of TMPMCT upon TDMAT and H 2 O exposure. In the DFT results in Fig. 2a , the molecular configuration of TMPMCT after adsorption indicates that the OMe ligands create bonds with the TiO 2 surface and the Cp(CH 3 ) 5 ligand faces the outer surface. Adsorption of TMPMCT on the TiO 2 surface is assumed to be dissociative adsorption via removal of individual OMe ligands as shown in Fig. 2a . A detailed description of the reaction mechanism is suggested in Supplementary Note 1 . The adsorption of TMPMCT can be considered facile, as it is exothermic and does not involve significant activation energy. Then, when the surface becomes saturated by adsorbed TMPMCT, the outer surface would become terminated by the Cp(CH 3 ) 5 ligands. These cyclopentadienyl ligands with low chemical reactivity [24] , [25] , [26] can then hinder the adsorption of subsequent TDMAT precursors. Fig. 2: Adsorption behaviour and blocking property of TMPMCT inhibitor. a Surface reaction energy diagram of TMPMCT molecules on the TiO 2 surface calculated by DFT. The structures below correspond to the Path 1. The dotted lines represent the reactions, where TS (transition states) structures were not calculated. Colours: Ti surf (light blue), Ti TMPMCT (yellow green), O surf (red), O TMPMCT (purple), C (brown), H (white pink). The corresponding chemical equations: Phy. : Cp(CH 3 ) 5 Ti(OMe) 3 , Ads. : *-Cp(CH 3 ) 5 Ti(OMe) 3 , 1OMe disso. : *-Cp(CH 3 ) 5 Ti(OMe) 2 + *-(OMe), 2OMe disso. : *-Cp(CH 3 ) 5 Ti(OMe) + 2·*-(OMe), 3OMe disso. : *-Cp(CH 3 ) 5 Ti + 3·*-(OMe). Phy. (Physisorption), Ads. (Adsorption), disso. (dissociation), surf (surface), * refers to adsorbed species. b WCA measurement with various exposure times of TMPMCT on the TiO 2 surface. Fitting of the JMAK model (dashed lines) to the data (points with error bars) obtained from c the growth of subsequent TiO 2 ALD on the TMPMCT inhibitor layer (20, 40 and 60 s), and d selectivity calculated from the thickness measured by ellipsometry. e Areal coverage of TMPMCT on the TiO 2 surface (10 nm × 10 nm) using various impingement numbers calculated by MC simulation and the coverage of TDMAT on the TMPMCT-inhibited surface. f Adsorption mechanism of TMPMCT inhibitor. Unoccupied sites serve as starting points for the nucleation sites of TiO 2 in subsequent ALD cycles. Source data are provided as a Source data file. Full size image Figure 2b shows the water contact angle (WCA) of the TMPMCT/TiO 2 surface as a function of TMPMCT exposure time. 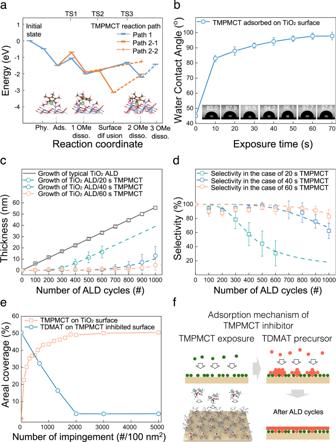Fig. 2: Adsorption behaviour and blocking property of TMPMCT inhibitor. aSurface reaction energy diagram of TMPMCT molecules on the TiO2surface calculated by DFT. The structures below correspond to the Path 1. The dotted lines represent the reactions, where TS (transition states) structures were not calculated. Colours: Tisurf(light blue), TiTMPMCT(yellow green), Osurf(red), OTMPMCT(purple), C (brown), H (white pink). The corresponding chemical equations: Phy.: Cp(CH3)5Ti(OMe)3, Ads.: *-Cp(CH3)5Ti(OMe)3, 1OMe disso.: *-Cp(CH3)5Ti(OMe)2+ *-(OMe), 2OMe disso.: *-Cp(CH3)5Ti(OMe) + 2·*-(OMe), 3OMe disso.: *-Cp(CH3)5Ti + 3·*-(OMe). Phy. (Physisorption), Ads. (Adsorption), disso. (dissociation), surf (surface), * refers to adsorbed species.bWCA measurement with various exposure times of TMPMCT on the TiO2surface. Fitting of the JMAK model (dashed lines) to the data (points with error bars) obtained fromcthe growth of subsequent TiO2ALD on the TMPMCT inhibitor layer (20, 40 and 60 s), anddselectivity calculated from the thickness measured by ellipsometry.eAreal coverage of TMPMCT on the TiO2surface (10 nm × 10 nm) using various impingement numbers calculated by MC simulation and the coverage of TDMAT on the TMPMCT-inhibited surface.fAdsorption mechanism of TMPMCT inhibitor. Unoccupied sites serve as starting points for the nucleation sites of TiO2in subsequent ALD cycles. Source data are provided as a Source data file. While the WCA of the hydrophilic TiO 2 surface [27] , [28] , [29] was 45.1° before exposure to TMPMCT, it rapidly increased to 83.0° and 97.7° after 10 s and 60 s exposure of TMPMCT, respectively. The increase in WCA is attributed to the formation of a chemically inert surface resulting from the Cp(CH 3 ) 5 Ti-ligand-terminated surface, as observed from the DFT results. No change of TiO 2 thickness was observed after the reaction between TMPMCT and H 2 O (see Supplementary Fig. 1e ), indicating TMPMCT is stable under H 2 O exposure. The blocking property of TMPMCT against 1000 cycles of ALD TiO 2 was evaluated at different TMPMCT exposure times. Figure 2c shows that TiO 2 growth on a TMPMCT-free surface is linear as a function of the ALD cycles. In contrast, there is almost no TiO 2 film growth on the 20 s TMPMCT inhibition layer, the growth exhibits linearity as in the TMPMCT-free sample after 200 cycles. The TiO 2 ALD film growth is inhibited for up to 700 and 900 cycles for the 40 s (blue points with error bars) and 60 s TMPMCT (orange points with error bars) inhibition layers, respectively. Then the TiO 2 ALD film growth is linear as in the case of 20 s TMPMCT inhibition layer. The selectivity is calculated from the thickness measured by ellipsometry (Fig. 2c ) and the results are shown in Fig. 2d . At small numbers of TiO 2 ALD cycles, the deposit amount significantly affects the selectivity. In addition, ellipsometry has errors in the scale of a few angstroms, resulting in large deviations in the calculated selectivity for low-thickness films. However, separate SEM and TEM results (Supplementary Fig. 2 ) revealed that there was almost no growth of the TiO 2 ALD thin film on 60 s TMPMCT/SiO 2 (Supplementary Fig. 2a ) and 60 s TMPMCT/10 nm TiO 2 /SiO 2 (Supplementary Fig. 2b ). 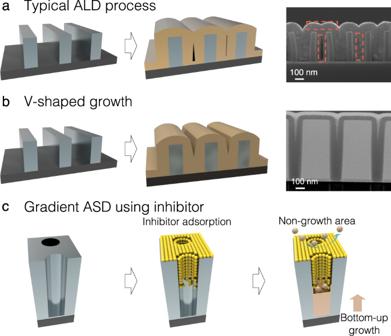Figure 2d indicates a very high calculated selectivity of >90% even after 900 cycles that is identical to the blocking of a 45-nm TiO 2 thin film. Fig. 1: Schematic illustrations of ASD processes for seamless gap-filling. aTypical ALD process.bALD process for V-shaped growth.cThe proposed gradient ASD process using an inhibitor. The inhibition of the TiO 2 film growth (using the same TDMAT precursor) herein was compared with that in the literature (Supplementary Table 1 ). The largest thickness of the inhibited TiO 2 film was 50 nm, achieved using a 43 nm poly(methylmethacrylate) inhibition layer [30] , followed by 48 nm, achieved using a 76 nm polynorbornene inhibition layer [7] . Comparatively, a single inhibitor layer was sufficient to inhibit the TiO 2 film growth to up to 45 nm in this study. Once the TiO 2 surface was exposed to TMPMCT, the OH-terminated TiO 2 surface changed to a Cp(CH 3 ) 5 Ti-terminated surface, and there was no significant reaction between the Cp(CH 3 ) 5 Ti-terminated surface and Ti precursors, as expected based on the DFT calculation (see Supplementary Fig. 3 ). The maximum blocking cycle increased with increasing TMPMCT exposure time. Interestingly, the nucleation of subsequent TiO 2 occurred over this specific cycle, leading to the degradation of the blocking property. Two possible reasons for this could be considered: (1) a direct reaction of the Cp(CH 3 ) 5 Ti-terminated surface and Ti precursor over a larger number of cycles and (2) the nucleation of TiO 2 on the defects in the TMPMCT inhibition layer. The DFT results eliminate the first reason. Therefore, we studied the nucleation of TiO 2 on the inhibited layer using the theoretical simulations and experimental approaches described below. Employing the previously-developed MC simulation, we investigated the physical adsorption and coverage of TMPMCT [8] , [12] , [31] by only considering the physical steric hindrance of TMPMCT on a surface and using the adsorption configuration from the DFT calculation. Figure 2e depicts the areal coverages of TMPMCT on the TiO 2 surface and TDMAT on the TMPMCT-inhibited surface. The area coverage of TMPMCT on the bare TiO 2 surface rapidly increases with increasing TMPMCT impingement (orange line) and reaches a plateau of ~50%. Therefore, the coverage of subsequent TDMAT on the TMPMCT-covered surface gradually decreases (blue line). Although the coverage of TMPMCT on the TiO 2 surface is saturated, some unoccupied adsorption sites remain. TMPMCT could not completely occupy the sites because of steric hindrance, and the TDMAT precursor can adsorb even on the TMPMCT-saturated surface (Supplementary Fig. 4 ). This result suggests that unoccupied sites, which are potential nucleation sites in the subsequent ALD process, exist even on the fully saturated TMPMCT layer. Therefore, the blocking property is degraded over specific cycles due to nucleation on unoccupied sites, as shown in Fig. 2f . This is consistent with our observations from Fig. 2 c and d. In addition, an interesting finding is that the number of unoccupied sites changed with increased exposure time at the beginning, which may explain the different blocking properties of the Ti inhibitor witnessed during different exposure times. Because TiO 2 nucleates only on the defects of the inhibition layer, island growth occurs based on the Volmer–Weber island growth mode in the subsequent ALD process [32] , [33] , [34] . To understand the degradation process quantitatively, we adopted a kinetic model based on the Johnson–Mehl–Avrami–Kolmogorov (JMAK) model [4] , [35] , [36] (details in Supplementary Note 2 , Supplementary Fig. 5 ). Based on the best fit results, the parameters including \(\,\dot{G}\) , \({\dot{N}}_{0}\) and v d are listed in Supplementary Table 1 , and the fitting results with the experimental data are plotted in Fig. 2 c and d (dashed lines). Figure 2c depicts an high goodness of fits for the thickness vs. ALD cycle number data of 0.933, 0.908 and 0.939 for 20 s, 40 s and 60 s of exposure time, respectively. Similarly, the selectivity data exhibits a highly consistent fit, as depicted in Fig. 2d . In addition, the nuclei density and nucleation growth of TiO 2 on the inhibited surface by 20 s, 40 s and 60 s TMPMCT were simulated using the JMAK model (Supplementary Table 2 and Supplementary Fig. 6 ). In fact, the defect of the inhibition layer is the OH-terminated original TiO 2 surface; hence, ALD TiO 2 easily nucleates on the defect sites during ALD if a defect site is still available. We assumed that the nucleation site density starts at 0 on the inhibition layer for JMAK simulation under ideal circumstances. Thus, the different nucleation site generation rates, \({\dot{N}}_{0}\) (presented in Supplementary Table 2 ) could be attributed to the different nucleation rates of TiO 2 caused by the different defect densities in the TMPMCT inhibitor layer. The higher defect density caused by shorter inhibitor exposure results in a higher nucleation site density and reflects faster nucleation than that of lower defect density samples. In addition, the number of nucleation delay cycles resulting from the fitting are 80, 620 and 800 cycles for 20, 40 and 60 s, respectively. In an ideal ALD process, the precursor chemisorbs onto the potential sites or surface. If the surface species or termination is not highly reactive towards the precursor, it should be converted to a high-reactivity surface termination during the following reactant exposure time. The time required for low-to-high-reactivity conversion of the surface may affect the nucleation delay. For instance, H-terminated Si surface is not highly reactive toward the adsorption of tetrakis(dimethylamino)-hafnium (TDMAH) precursor; however, the surface can be converted to a OH-terminated Si surface via H 2 O counter reactant exposure or an O-terminated Si surface via O 3 reactant pulsing, which exhibits high reactivity towards the TDMAH precursor [37] . In this study, this reason can be ruled out because the potential adsorption site for the next TDMAT precursor is the defect site, which is also the original TiO 2 surface. When a TMPMCT inhibitor is used, the coverage of TMPMCT limits the potential adsorption site of the next TDMAT precursor, forming a sub-monolayer after each cycle. The time required for monolayer formation from a sub-monolayer can drive the nucleation delay. Thus, the slower nucleation rate observed on the longer-TMPMCT exposure sample leads to the longer nucleation delay, as simulated. A theoretical interpretation of the experimental results suggests that the control of unoccupied sites, which are the same as defect sites, is the most important factor for a higher blocking property. The DFT results showed that the TMPMCT chemisorbs onto the TiO 2 surface by releasing OMe ligands, but not all OMe ligands are dissociated. If the OMe ligand could also be eliminated, additional space would be available for the formation of the inhibitor, as depicted in Fig. 3a . Although the TMPMCT is not fully oxidised to TiO 2 by an H 2 O reactant because of the remaining Cp(CH 3 ) 5 ligands, H 2 O can further eliminate the OMe ligands through a hydrolysis reaction with the adsorbed TMPMCT [38] . The DFT calculation modelled a reaction of H 2 O molecules with OMe ligands of the adsorbed TMPMCT and releases MeOH by-product, resulting in the formation of Cp(CH 3 ) 5 Ti(OMe) 3-x (OH) x (x = 0, 1, 2 and 3). The energy for the ligand–exchange reaction between OMe and OH from H 2 O on the surface according to the number of H 2 O molecules is presented in Fig. 3b . Two adsorption configurations are considered due to a large degree of freedom, Config A and Config B. Both configurations show a decrease in E ad as the more OMe ligands are modified into OH. From MC simulations for the adsorption of Cp(CH 3 ) 5 Ti(OMe) 3-x (OH) x molecules, the results, shown in Fig. 3c , indicate that the point coverage of Cp(CH 3 ) 5 Ti(OMe) 3-x (OH) x increased from 6.0% (without additional H 2 O and remaining 3OMe ligands) to 6.6%, 6.9% and 7.2% while eliminating 1OMe, 2OMe and 3OMe ligands, respectively. Thus, from the theoretical calculations, an additional H 2 O pulse can create more space for additional inhibitor adsorption, increasing the inhibitor coverage and decreasing the defect sites. Fig. 3: Blocking property of TMPMCT with an additional H 2 O pulse. a Schematic of TMPMCT exposure with an additional H 2 O pulse to improve coverage. b Adsorption energy of hydrolysed TMPMCT species, Cp(CH 3 ) 5 Ti(OMe) 3-x (OH) x (x = 0, 1, 2 and 3), calculated by DFT. c MC simulation results for the adsorption of Cp(CH 3 ) 5 Ti(OMe) 3-x (OH) x with steric hindrance in cases x = 1, 2 and 3. Fitting of the JMAK model to data (points with error bars) obtained from d growth and e selectivity in the case of 20 s TMPMCT with and without additional H 2 O pulse samples. Fitting of the JMAK model to data (points with error bars) obtained from f growth and g selectivity in the case of 40 s TMPMCT with and without additional H 2 O pulse samples. Source data are provided as a Source data file. Full size image We modified the single 20 s TMPMCT pulse into two 10 s TMPMCT pulses disrupted by a 2.5 s pulse of H 2 O and the single 40 s TMPMCT pulse into two 20 s TMPMCT pulses disrupted by a 5 s pulse of H 2 O (Supplementary Fig. 7 ). We then evaluated their blocking properties up to 1000 cycles of ALD, as shown in Fig. 3 d– g . As shown in Fig. 2 , the TiO 2 growth was inhibited for up to 200 and 700 cycles under 20 s and 40 s TMPMCT exposure conditions, respectively. With additional H 2 O exposure, however, the TiO 2 growth was inhibited for up to 400 and 900 cycles for 20 s and 40 s samples, respectively, as shown in Fig. 3 d– g . The fitting results with the JMAK model showed high goodness of fits as shown in Fig. 3 d– g . 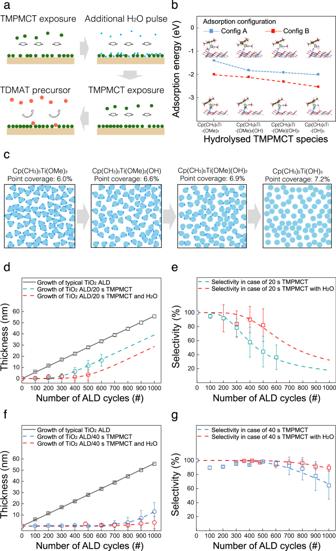Fig. 3: Blocking property of TMPMCT with an additional H2O pulse. aSchematic of TMPMCT exposure with an additional H2O pulse to improve coverage.bAdsorption energy of hydrolysed TMPMCT species, Cp(CH3)5Ti(OMe)3-x(OH)x(x = 0, 1, 2 and 3), calculated by DFT.cMC simulation results for the adsorption of Cp(CH3)5Ti(OMe)3-x(OH)xwith steric hindrance in cases x = 1, 2 and 3. Fitting of the JMAK model to data (points with error bars) obtained fromdgrowth andeselectivity in the case of 20 s TMPMCT with and without additional H2O pulse samples. Fitting of the JMAK model to data (points with error bars) obtained fromfgrowth andgselectivity in the case of 40 s TMPMCT with and without additional H2O pulse samples. Source data are provided as a Source data file. From the parameters obtained from the fittings (Supplementary Table 3 ), the decrease in the nucleation site generation rate, \({\dot{N}}_{0}\) , and the increase in the nucleation delays, v d , reflect an increase in the TMPMCT coverage by addition H 2 O, which leads to the reduction of defect sites, as predicted by DFT calculations and MC simulations. From the results, we investigated different inhibitor coverages in a deep nanoscale hole pattern. We performed experiments on 8-inch wafers in a spatially divided ALD system, which has a high-volume manufacturing capability (Supplementary Fig. 8 ). We used 730 cycles of ALD on this nanoscale hole pattern to form a 40 nm thick TiO 2 layer, based on the growth per cycle (GPC) of TiO 2 . As shown in Fig. 4a , while the hole deposited by TiO 2 without TMPMCT almost was closed off with the formation of a seam, no pinch-off was observed for 40 s and 60 s TMPMCT exposure samples. The gradient blocking property was consistent for other sampling points in the same 8-inch wafer (TEM images in Supplementary Fig. 9 ). The thicknesses of TiO 2 on the 40 s sample were distributed from 10 nm to 30 nm (blue points in Fig. 4b ). The thicknesses of the 60 s sample were distributed more widely, from 2 nm to 30 nm with changing depth (orange points in Fig. 4b ). In addition, the 40 s TMPMCT with H 2 O samples exhibited a thickness distribution similar to that of the 60 s TMPMCT sample without H 2 O. Near the opening, the blocking property of the longer exposure sample was more significant than that of the shorter exposure sample, similar to those on planar samples. The selectivity (Fig. 4c ) of the 60 s sample was almost 90% at the top of the hole but decreased to 20% with increasing depth. The two 40 s samples with and without H 2 O also exhibited selectivity changes. Fig. 4: Hole pattern with a depth of 1600 nm, an opening diameter of 100 nm and a bottom diameter of 50 nm used for gap-filling. a TEM images of the subsequent 40 nm thick TiO 2 ALD film on the 0, 40 and 60 s TMPMCT inhibitors and 40 s TMPMCT with an additional H 2 O/10 nm TiO 2 /SiO 2 hole. b Growth and c selectivity calculated from the TEM results. d Relative coverage of various TMPMCT pulses, as calculated from the equation described in Supplementary Note 3 and depicted in illustrations e 40 s TMPMCT pulse, f 60 s TMPMCT pulse. Source data are provided as a Source data file. Full size image Because 3D nanostructures possess a much larger surface area than 2D planar surfaces, the adsorption behaviour on both structures should be different under the same exposure conditions, leading to different molecular adsorption densities. To quantify the results, we adopted a kinetic model to estimate the adsorption density of TMPMCT inside 3D nanoscale holes. The time t (s), which is required to cover the surface area of a 3D hole down to the depth λ (nm) can be calculated by the following equation (details in Supplementary Note 3 ) [39] : 
    t=∫_0^tdt=Q√(2πmkT)/Pp/A_hole∫_0^Ldλ(1+3pλ/16A_hole)
 Although a perfectly cylinder-shaped hole was not used for this experiment, it can provide a good explanation for the approximate adsorption density changes. 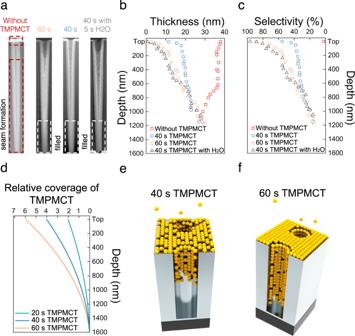Fig. 4: Hole pattern with a depth of 1600 nm, an opening diameter of 100 nm and a bottom diameter of 50 nm used for gap-filling. aTEM images of the subsequent 40 nm thick TiO2ALD film on the 0, 40 and 60 s TMPMCT inhibitors and 40 s TMPMCT with an additional H2O/10 nm TiO2/SiO2hole.bGrowth andcselectivity calculated from the TEM results.dRelative coverage of various TMPMCT pulses, as calculated from the equation described in Supplementary Note3and depicted in illustrationse40 s TMPMCT pulse,f60 s TMPMCT pulse. Source data are provided as a Source data file. Figure 4d shows a plot of relative coverage of TMPMCT with different pulses versus the hole depth, calculated from the above-mentioned equation. The molecular adsorption on the top area is faster than that inside the hole because more time is required for molecules to reach the lower portion of the hole (Fig. 4e , f ). Therefore, the relative coverage of TMPMCT was the highest at the top (depth = 0 nm) and decreased with increasing depth for all TMPMCT pulses. The longest TMPMCT pulse, 60 s, resulted in higher relative coverage at the top than the 40 s and 20 s TMPMCT pulses. As a result, the application of a short TMPMCT pulse would narrow the relative-coverage distribution. Therefore, more exposure time is required to cover a surface deeper inside the hole because of the geometrically limited flux of the inhibitor molecule. In other words, under constant exposure conditions, the adsorption density of TMPMCT should change with the changing depth, as plotted. Because the adsorption density of TMPMCT is proportional to the blocking property and selectivity, the relative coverage as a function of depth should be similar to the selectivity as a function of depth. Compared with Fig. 4c , plots resulting from the kinetic model demonstrate a high consistency, indicating that the blocking property changes depending on geometrical factors. Based on this interpretation, we also performed a gradient ASD for seamless deposition on 8-inch wafers in a production-scale system (Supplementary Fig. 8 ). 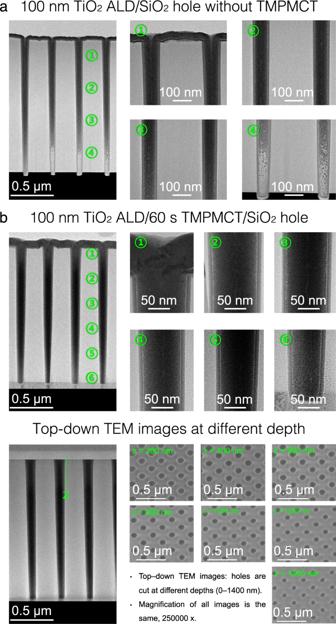Fig. 5: 100 nm TiO2ALD deposited in holes with and without TMPMCT inhibitor. aCross-sectional TEM images of the hole pattern (depth = 1600 nm) for 100 nm TiO2ALD without TMPMCT. Unfilled zones are observed at the bottom (zone 4), and seam formation occurs along the centreline of the hole (zones 2 and 3).bCross-sectional TEM images of the 100 nm TiO2ALD/60 s TMPMCT/SiO2hole and top-down TEM images at different depths, demonstrating hole filling without any seam formation. Figure 5a indicates that it is not feasible to fill the high-aspect-ratio hole (depth = 1600 nm) perfectly using 100 nm TiO 2 ALD without TMPMCT. Cross-sectional TEM images show an unfilled zone and seam formation along the centreline of the hole. In addition, the seam formation significantly varied with the position in the wafer; thus, large voids were observed in the non-uniform regions of the wafer (TEM image in Supplementary Fig. 10 and uniformity data in Supplementary Table 4 ). Furthermore, when 60 s TMPMCT was used, perfect filling was observed without any seam or void formation, as shown in the cross-sectional and top-down TEM images acquired at different depths (Fig. 5b ). Energy-dispersive spectroscopy (EDS) mapping (Supplementary Fig. 11 ) revealed that only Si, Ti and O were present without any significant amount of C. In addition, the results of the EDS line profile across the ASD TiO 2 /TMPMCT/SiO 2 hole sample (Supplementary Fig. 12 ) demonstrate that no significant carbon impurities were left by TMPMCT between the substrate and TiO 2 , even after the cessation of the blocking property (Supplementary Fig. 12b ). TMPMCT should exist in a Cp(CH 3 ) 5 Ti form after ASD TiO 2 (DFT results in Fig. 2a ), forming Ti–C impurities; however, only a negligible amount of C was detected within the limits of the measurement (Supplementary Fig. 12d ). Fig. 5: 100 nm TiO 2 ALD deposited in holes with and without TMPMCT inhibitor. a Cross-sectional TEM images of the hole pattern (depth = 1600 nm) for 100 nm TiO 2 ALD without TMPMCT. Unfilled zones are observed at the bottom (zone 4), and seam formation occurs along the centreline of the hole (zones 2 and 3). b Cross-sectional TEM images of the 100 nm TiO 2 ALD/60 s TMPMCT/SiO 2 hole and top-down TEM images at different depths, demonstrating hole filling without any seam formation. Full size image We proposed a Ti precursor inhibitor, TMPMCT, and studied its chemical and physical adsorption behaviour by using theoretical methods, DFT and MC simulations. The degradation of the TiO 2 blocking property with an increasing number of ALD cycles was investigated by adopting an MC simulation and a kinetic growth model, the JMAK equation. It was revealed that the unoccupied sites in the inhibitor layer play an important role in the degradation of ASD TiO 2 films, and the blocking property could be controlled by adjusting the surface coverage of the inhibitor. To improve the blocking property, an additional H 2 O pulse was added, as suggested by theoretical calculations and evaluation by DFT and MC simulation. H 2 O was found to eliminate the OMe ligands of the adsorbed TMPMCT, creating more space for additional adsorption of TMPMCT. A monolayer of the TMPMCT inhibitor was found to block a 45 nm thick TiO 2 thin film in the subsequent ALD process, which is the thickest film thickness ever reported to date. In addition, the TMPMCT inhibitor with an H 2 O pulse demonstrated a significantly improved blocking property up to 49 nm of TiO 2 blocking. In 3D nanoscale hole patterns, ASD TiO 2 films exhibited a geometrically anisotropic growth. By adopting a kinetic model, the adsorption behaviour of a TMPMCT inhibitor inside 3D holes was interpreted. The adsorption density of the inhibitor was found to vary inside the 3D holes because of the geometrically limited flux, leading to a gradient ASD. A perfectly seamless TiO 2 deposition was obtained in the nanoscale 3D holes through ASD. Because the gradient ASD process works based on the fundamentals of molecular chemical and physical behaviours, this approach can be applied to other material systems in ALD. In addition, the experiments were repeated many times with a large number of samples on a production-scale system. The results were used for plotting graphs; parameters such as thickness and selectivity were averaged from different runs, and their standard deviations were determined (Supplementary Table 4 and Supplementary Fig. 14 ). The gradient ASD approach proposed herein has high reliability because it can be reproduced and applied to a large-scale ALD system. Hence, the fundamental understandings derived from this study can be directly applicable at manufacturing scales. Sample preparation Experiments were conducted on a lab-scale ALD machine (Atomic-Shell, CN1 Co., Korea) and scaled to a high volume production by a spatial-divided ALD (SALD) machine at the Samsung Advanced Institute of Technology. The SALD system includes an 8-inch rotary chamber that features a 16-split shower head with individual nozzle control. The susceptor rotates at 40 rpm, and the chamber can load three 8-inch wafers simultaneously, as shown in Supplementary Fig. 8 . In the lab-scale ALD system, a small coupon wafer was loaded, and the precursor and counter-reactant were dosed on to the wafer via a nozzle line. Additional information on the lab-scale ALD system can be found in refs. 12 , 40 , 41 . The TiO 2 precursors, titanium isopropoxide (TTIP) (Sigma-Aldrich) and tetrakis-(dimethylamido)titanium (TDMAT) (Oceanbridge Co., Ltd, Korea), were contained in a canister at 50 °C. The H 2 O reactant was kept at 25 °C. Trimethoxy-(pentamethylcyclopentadienyl)titanium(IV) (Cp(CH 3 ) 5 Ti(OMe) 3 ), abbreviated as TMPMCT (Ichems Co., Korea), was used as an inhibitor and was investigated at different temperatures. The substrates used in these experiments included a planar SiO 2 wafer and hole patterns (1600 nm depth, 100 nm diameter opening, 50 nm bottom diameter). They were sequentially cleaned using acetone, isopropyl alcohol and deionised water and dried using N 2 flow. All experiments were performed at 180 °C [42] , [43] , [44] , [45] , [46] . The GPCs were approximately 0.40 and 0.55 Å/cycle for TTIP and TDMAT precursors, respectively (Supplementary Fig. 1a–d ). The adsorption mechanism of the TMPMCT inhibitor on the TiO 2 surface was investigated at different adsorption times (20–60 s) and canister temperatures (70–100 °C) (Supplementary Fig. 1e and f). The adsorption mechanism of the TMPMCT inhibitor on various substrates, namely, TiO 2 -deposited SiO 2 , Ru-deposited SiO 2 , HfO 2 -deposited SiO 2 , TiN and SiO 2 , was also investigated; the results are shown in Supplementary Fig. 1g . The TMPMCT inhibitor layer was used to evaluate the blocking property against TiO 2 ALD on SiO 2 and 10 nm TiO 2 -deposited SiO 2 substrates, as shown in Supplementary Fig. 2 . The results show that the TiO 2 ALD thin films were obtained on the bare surfaces, but no TiO 2 growth was observed on the TMPMCT-inhibited surfaces. The blocking property of the TMPMCT was examined at 20, 40 and 60 s exposure on TiO 2 -deposited SiO 2 substrate, against 1000 cycles of TiO 2 ALD. An additional H 2 O pulse was included to improve the coverage and blocking property of TMPMCT by inserting an H 2 O pulse to interrupt the continuous TMPMCT pulse. The sequence followed was TMPMCT pulse–additional H 2 O pulse–TMPMCT. In the gradient ASD experiments, we used an SiO 2 hole pattern with a 1600 nm depth, 100 nm opening diameter and 50 nm bottom diameter. Before TMPMCT exposure, a 10 nm TiO 2 was deposited on the SiO 2 hole patterns to produce a TiO 2 surface; hence, the opening diameter was reduced from 100 nm to 80 nm. We then investigated 20, 40 and 60 s of TMPMCT exposure and 40 s of TMPMCT with H 2 O pulses in the gap-filling processing of 40 nm and 100 nm TiO 2 . Sample characterization The thickness of the deposited films was measured using field-emission scanning electron microscopy (FE-SEM; JEOL JSM-7001F; JEOL, Ltd.), which included ellipsometry at an incidence angle of 64.885° for thicknesses between 245 and 1000 nm (i.e., from −1.24 to 5.06 eV), and high-resolution transmission electron microscopy (JEM-2100F, JEOL) equipped with an energy-dispersive X-ray spectroscopy and a 50 nm 2 probe (solid angle = 0.28 sr, take-off angle = 24.1°), as shown in Figs. 4 , 5 , and Supplementary Figs. 9 , 10 , 11 , 12 . Theoretical calculations DFT calculations were performed using the Vienna ab initio simulation package version 5.4.4 [47] . Within the DFT + U framework, the Perdew–Burke-Ernzerhof generalised gradient approximation functional was employed to treat the exchange-correlation energy [48] while applying the D3(BJ) dispersion correction [49] . Using Dudarev’s approximation [50] , parameter U eff (=U − J) for Ti was set to 3, which is an optimised value from the literature [51] . A clean anatase TiO 2 (101) surface was used to simulate surface reactions. ALD-grown TiO 2 was reported to exist in the anatase phase at a considered temperature in this study [41] , [52] , and the lowest surface energy was in the (101) plane [53] . Most H 2 O and OH moieties desorb from the anatase TiO 2 (101) surface at temperatures above 400 K [54] . The first surface model, a three-layered TiO 2 surface with dimensions of 10.5 × 11.4 × 28 Å, was used to locate local or global minimum structures while the forces acting on the atoms were less than 0.02 eV Å −1 . Energy barriers were obtained via the nudged elastic band method with a force tolerance of 0.05 eV Å −1 [55] , [56] . The Cp(CH 3 ) 5 Ti-terminated surface was simulated using the second surface model, two-layered TiO 2 surface (20.9 × 11.4 × 28 Å), with a force tolerance of 0.02 eV Å −1 . The surface models contained more than 10 Å of the vacuum region. All calculations were conducted with an energy cut-off level of 500 eV. A 2 × 2 × 1 k-point grid for the surface models was set according to the Monkhorst–Pack scheme after convergence test. The adsorption energy (E ad ) was defined as E ad = E total − (E slab + E molecule ), where E total and E slab are the total electronic energies of the slab with and without an adsorbate, respectively, and E molecule is the energy of the gaseous molecule. The physical adsorption, the coverage of TMPMCT on the TiO 2 surface, and the elimination of OMe ligands of TMPMCT using H 2 O were investigated via MC simulations. The MC simulations were performed using a modified algorithm, which was run on the simulation programme “R” (version 3.6.1; GUI 1.70; EL Capitan build 7684). Further information can be found in our previous reports [8] , [12] (algorithm in Supplementary Fig. 13 ). We also employed the Johnson–Mehl–Avrami–Kolmogorov (JMAK) model to quantify the blocking property and degradation with experimental data [4] , [35] , [36] . The JMAK model was calculated using the Matlab software (Matlab R2018b version 9.5). In addition, the adsorption density of TMPMCT inside a 3D nanoscale hole was calculated using various TMPMCT pulses of 20, 40 and 60 s.